The cavefish genome reveals candidate genes for eye loss Natural populations subjected to strong environmental selection pressures offer a window into the genetic underpinnings of evolutionary change. Cavefish populations, Astyanax mexicanus (Teleostei: Characiphysi), exhibit repeated, independent evolution for a variety of traits including eye degeneration, pigment loss, increased size and number of taste buds and mechanosensory organs, and shifts in many behavioural traits. Surface and cave forms are interfertile making this system amenable to genetic interrogation; however, lack of a reference genome has hampered efforts to identify genes responsible for changes in cave forms of A. mexicanus. Here we present the first de novo genome assembly for Astyanax mexicanus cavefish, contrast repeat elements to other teleost genomes, identify candidate genes underlying quantitative trait loci (QTL), and assay these candidate genes for potential functional and expression differences. We expect the cavefish genome to advance understanding of the evolutionary process, as well as, analogous human disease including retinal dysfunction. Some of the most fundamental questions in evolutionary biology involve how organisms can adapt to new environments. Natural populations under strong selection may be especially useful in deciphering the genetic variants underpinning these evolutionary responses. Yet, few systems possess dramatic phenotypic changes that can be definitively attributed to selection pressures of a new environment. Even fewer species can be used to understand how evolution proceeds when repeated in separate populations. Cave animals offer one of the most exciting systems in which to study these questions [1] . Specifically, surface forms of the Mexican tetra, Astyanax mexicanus , colonized multiple caves in northeastern Mexico and evolved extreme cave-associated traits at least four independent times over the past 2–3 Myr (refs 2 , 3 ). Cavefish populations exhibit repeated morphological evolution for a variety of traits including eye degeneration [2] , [4] , pigment loss [5] , [6] , increased size and number of specialized mechanosensory organs called neuromasts [7] and increased numbers of taste buds [4] . Cavefish have also evolved behavioural differences relative to their surface-dwelling counterparts including increased attraction to vibrations [7] , increased olfactory capabilities [8] , altered feeding angles [9] and loss of schooling and aggression [10] , [11] . Further, cavefish lose body weight less quickly than surface morphs [8] and show dramatic sleep reductions compared to surface fish [12] . The polarity of these trait changes is known (derived in cavefish). Therefore, these natural replicates offer a unique opportunity to study the genetic bases of parallel and convergent evolutionary changes [1] . Further, A. mexicanus is amenable to molecular genetic manipulation in the lab [13] , [14] , and prior QTL (quantitative trait locus) analyses of surface and cavefish crosses identified genomic regions regulating numerous behavioural and morphological traits [4] , [7] , [8] , [9] , [10] , [15] . In this work, we present the first de novo genome assembly for A. mexicanus cavefish to allow for more precise identification of candidate genes underlying QTL than was previously possible with syntenic comparisons to zebrafish [15] , [16] . We demonstrate the effectiveness of this approach by identifying candidate genes for eye development and other cave-derived traits. We further analyze RNAseq data to survey these candidate genes for potential coding and expression level differences between the surface and cave populations. For many traits, we expect that the cavefish genome will provide a tool for discovery of the role of individual genes and pathways. Sequencing and annotation The sequenced cavefish individual was the first-generation offspring of two wild-caught parents, which originated from Pachón cave, Tamaulipas, Mexico. While there are at least 29 caves that contain Astyanax cavefish, the Pachón cavefish are the most studied and exhibit the most extreme troglomorphic phenotypes relative to the other caves [2] . This genome draft was assembled to a size of 964 Mb, which is similar in size to a congeneric in Brazil [17] . The draft genome contains 10,735 scaffolds (N50 contig=14.7 kb; N50 scaffold=1.775 Mb), and the longest scaffold size was 9.823 Mb ( Supplementary Data 1 ). Using the Ensembl annotation pipeline [18] and RNAseq transcript evidence (eight unique tissues; Supplementary Data 2 ), we predicted a total of 23,042 protein-coding genes, similar to other sequenced teleost fishes. Zebrafish is the closest sequenced relative to cavefish (diverged approximately 250 Myr) [19] , and we annotated 16,480 one-to-one orthologs with zebrafish. To estimate gene representation in the draft genome, we used assembled cavefish transcripts and evolutionarily conserved gene models. Alignment of the Astyanax best open reading frames ( Supplementary Data 2 ) to the genome scaffolds found that across tissue-specific transcriptomes, a median of 81% of transcripts align over at least 75% of their length with at least 90% identity. Further, CEGMA analyses [20] indicated that 95% of the 248 ultra-conserved core eukaryotic genes are present in the genome assembly, and 69% of the 248 ultra-conserved core eukaryotic genes were considered complete genes. Collectively, this suggests that the assembly has captured much of the protein-coding sequence in the cavefish genome. Transposable element annotation One-third of the cavefish genome is composed of transposable elements (TEs) ( Supplementary Data 3 and 4 ). This repetitive content is comparable to most published fish genomes ( Supplementary Data 3 ), with the exceptions of zebrafish (52.2% TEs) [21] and Fugu (2.8%) (ref. 22 ). In the cavefish, DNA transposons are more abundant and diversified than retrotransposons, as there are at least 12 different superfamilies of DNA transposons representing 12.7% of the genome. In contrast, retrotransposons comprise only 2.3% of the genome ( Supplementary Data 4 ). It appears that a recent wave of transposition occurred in the cavefish genome ( Fig. 1 ) and was composed mostly of Tc-Mariner and hAT superfamilies, which currently comprise approximately 9.5% of the cavefish genome. Similarly, zebrafish experienced a recent large expansion of repeat families, including Tc-Mariner and hAT superfamilies, whereas another common model, stickleback, has not (RepeatMasker Genomic Datasets). We estimated the potential age of the different of copies for each TE-related superfamilies by calculating Kimura distances assuming that most of the mutations in TE copies are neutral. The rates of transversions ( q ) and transitions ( p ) were transformed in Kimura distances using [ K =−½ ln( 1 − 2p − q )− ¼ ln( 1 − 2q )]. The cavefish genome differs in comparison with zebrafish in that it appears to lack very young elements (as indicated by the Kimura distance from the consensus, Fig. 1 , RepeatMasker Genomic Datasets). Given the caveats of possible assembly artefacts, lack of very young elements indicates that it is unlikely that many copies of Tc-Mariner and hAT superfamilies are still active in the cavefish genome (confirmed by analyses of transcriptomes, Supplementary Data 5–9 ). 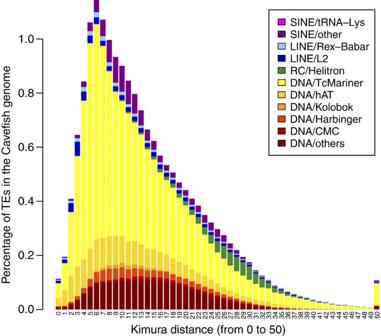Figure 1: TE superfamilies’ history in the cavefish genome. Only superfamilies that show content higher than 0.1% inSupplementary Data 4were used. Kimura distances are ranged from value 0 representing recent TE copies to 50 for the old TE insertions. Figure 1: TE superfamilies’ history in the cavefish genome. Only superfamilies that show content higher than 0.1% in Supplementary Data 4 were used. Kimura distances are ranged from value 0 representing recent TE copies to 50 for the old TE insertions. Full size image Identification of candidate genes under QTL Perhaps the most distinct trait in cavefish is the reduced, nearly absent eye ( Fig. 2 ), which is independently derived in multiple, independent cave invasions [2] , [3] , [23] . In cavefish, early eye development is largely similar to the eye development in surface fish in that lens vesicles and optic cups form, albeit, they are smaller in cavefish even at very early stages (14 h.p.f., hours post fertilization [24] ). The lens apoptosis begins after 25 h.p.f. (refs 24 , 25 ), and the retina undergoes significant apoptosis at about 35 h.p.f. (ref. 24 ). This apoptosis continues for days to weeks, and leads to an arrest of eye development [25] , [26] . We examine the genome for genes under QTL for eye size from Pachón cavefish × surface fish crosses from various studies [4] , [6] , [7] , [8] , [15] , [16] . 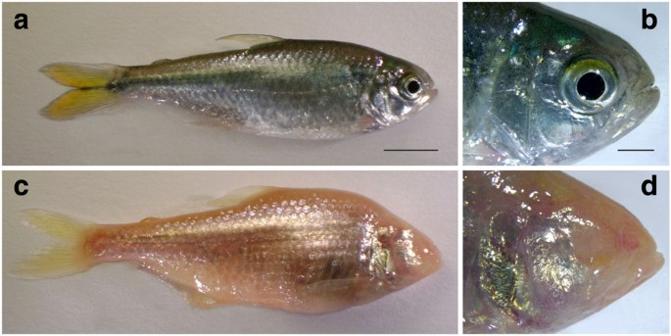Figure 2: Photographs of surface and cavefish. (a,b) Surface fish (line 152) (c,d) Pachón cavefish (line 45). Scale bar fora,cis 1 cm. Scale bar forb,dis 0.25 cm. Photos by B.A.S. Figure 2: Photographs of surface and cavefish. ( a , b ) Surface fish (line 152) ( c , d ) Pachón cavefish (line 45). Scale bar for a , c is 1 cm. Scale bar for b , d is 0.25 cm. Photos by B.A.S. Full size image Across studies, we count a total of 15 non-overlapping QTL for eye-related phenotypes discovered in the Pachón population [4] , [7] , [8] , [9] , [10] , [15] , [16] ( Supplementary Fig. 1 ). Scaffolds often did not span the entire critical region comprising a QTL; thus, each QTL critical region may be distributed across several scaffolds. All genes on a scaffold containing a marker linked to the QTL were included. In total, 2,408 genes out of the 23,042 genes annotated in this draft of the genome were associated with these genomic regions. It is likely that a significant portion of these genes that are physically linked to the causal variant are not responsible for the phenotype. To narrow the list of candidate genes, we examined the gene expression in surface and cave populations with a developmental time course taken at 10 h.p.f., 24 h.p.f., 1.5 days post fertilization (d.p.f. ), and 3 d.p.f. RNA from each time period was extracted from 50 whole, pooled individuals and Illumina reads were generated for cavefish and surface fish pools separately. An important caveat to interpreting the gene expression data is that even early in development, cavefish eyes are smaller than surface fish eyes, and lower numbers of transcripts may reflect smaller eyes and not necessarily downregulation. The transcript sequences were also used for obtaining coding variant differences between surface fish and cavefish. Due to the enormity of defining gene to QTL associations for many troglomorphic traits, we primarily focused on the eye phenotype. Here we used expression data and integrated pathway analysis [27] to predict likely phenotypes and the genes potentially underlying those phenotypes. Utilizing prior knowledge of predicted outcome between transcriptional regulators and their target genes [27] , we implicate 30 genes under the QTL to result in congenital eye anomalies. The direction of gene expression change between surface fish and cavefish supports an increased likelihood of eye anomalies in cavefish relative to surface fish at 10 h.p.f., 24 h.p.f., and 1.5 d.p.f. (for example, 12/27, 12/19, 11/30 genes have expression direction consistent with increased congenital anomaly of the eye, respectively; biased-corrected z score ≥2.266, P <0.0001 in all cases, see ref. 27 for details of z score calculation). At the last sampled time point (3 d.p.f. ), the expression data are consistent with increased cavefish eye anomalies, but interestingly, the z scores become smaller with the progression of development ( Supplementary Data 10–16 ) and are not significant at 3 d.p.f. We performed an enrichment test with data combined across time points and found that the QTL were enriched for genes involved in congenital anomaly of the eye, (30/1,560 relative to 159/12,040 in the total expression data set; χ 2 -test with Yates correction P value <0.034, χ 2 =4.48, odds ratio=1.57, 95% confidence interval of odds ratio=1.05–2.35). Additional genes involved in eye development, function and disease were enriched in the QTL set, though not significantly so (129/1,560 relative to 921/12,040 in total data set; χ 2 -test with Yates correction P value=0.35, χ 2 =0.88, odds ratio=1.10, 95% confidence interval of odds ratio=0.91–1.34). Therefore, we contend that the eye-related QTL are qualitatively enriched for eye-related genes relative to the rest of the genome, but the eye-related QTL are quantitatively more likely to contain genes associated with congenital eye defects. Specific candidate genes under eye-related QTL Several genes found under the QTL are classic candidates for eye development, and we highlight several, which may be particularly promising. We narrowed down the list of candidate genes under the QTL by focusing on those with expression differences between cavefish and surface fish. Statistical comparisons of gene expression levels were performed using the measure of log fold change performed in Cuffdiff 2.1.0 (ref. 28 ) (see Cuffdiff 2.1.0 documentation for additional details of test). Unless otherwise noted, all P values given below for differential expression between cave and surface fish were generated by this test. Linkage group (LG) names are inconsistent across studies; thus, the LGs given below correspond to the naming scheme in the original study in which the QTL was found and those studies are cited after the LG name. One of these candidate genes identified by this method is cryaa , an antiapoptotic chaperone protein whose absence of gene expression was hypothesized to play a role in cavefish eye degeneration [26] . Cryaa falls under a QTL for eye size on LG 27 (scaffold containing marker Am229b) from Protas et al . [4] Next, pitx3 is essential for lens development in zebrafish [29] , [30] and knockdown experiments result in zebrafish with degenerate lens and retinas and misshapen lower jaws [29] . Cavefish exhibit significantly lower expression of pitx3 at 24 h.p.f. and 3 d.p.f. ( P <0.002 at both time points, qualitatively lower at all times), but there are only two synonymous differences between surface and cavefish pitx3 . Pitx3 is located under the QTL for lens length on LG14 (ref. 4 ) and for eye size on LG4 (ref. 7 ). Similarly, rx3 is located under a QTL for eye size on LG4 (refs 4 , 8 ) and underlies a loss of eyes in zebrafish ( chokh ) and medaka ( eyeless ) mutants [31] , [32] . Rx3 exhibits significantly less expression in cavefish than in surface fish at 10 h.p.f. and 3 d.p.f. ( P <0.0003 at both time points, qualitatively lower at all times) and no coding variants. Likewise, under the QTL for eye size on LG4 (refs 4 , 8 ) are the genes olfm2a and olfml2a. Zebrafish knockdowns of olfm2 result in abnormalities in the olfactory pits, eyes and optic tectum as well as reduced and less-defined Pax6 expression in the eye [33] , and olfm2a exhibited significantly lower expression in cavefish at 3 d.p.f. ( P <0.001). We did not detect coding differences in olfm2a , and data were unavailable for olfml2a. Lastly, BCoR is found on LG19 (refs 4 , 8 ). BCoR is linked with ocular colobomas in human and zebrafish [34] and its binding partner, BCL6, has been shown to control optic cup morphogenesis through regulation of p53 in zebrafish [35] . Cavefish exhibit significantly lower expression of BCoR at 10 h.p.f. ( P <0.013), and four nonsynonymous coding differences exist between surface and cavefish, though all appear to be in evolutionary labile sites. Importantly, these genes represent only a subset of the interesting candidates under QTL. Candidate genes in QTL with potentially pleiotropic effects For several QTL, multiple troglomorphic phenotypes co-localize with eye size, and this co-localization has been suggested as an evidence that selection for some cave-adapted traits resulted in pleiotropic degeneration of eyes [7] . One of these QTL is involved in vibration attraction behaviour, eye size and superficial neuromast number at the orbit on LG2 (ref. 7 ). This same QTL for eye size has been identified in multiple studies (LG7 (ref. 4 ), LG8 (refs 4 , 8 ) and LG1 (ref. 16 )) and a QTL for the thickness of the inner nuclear layer of the retina on LG2 (ref. 15 ). These LGs from various studies all correspond to the same genomic region, and here we count this region as a single QTL. We mainly concentrate on genes that are expressed in both cave and surface fish and appear to have not been pseudogenized in cavefish, as these are genes most likely to have pleiotropic effects and to be good candidates for driving multiple phenotypes that co-localize to the same QTL. One of the more interesting candidate genes in this region is shisa2 , which inhibits Wnt and fibroblast growth factor signalling by retaining their respective receptors, Frizzled and fibroblast growth factor receptor, in the endoplasmic reticulum [36] . Cavefish expression of shisa2 is qualitatively higher than surface fish at all time points (significantly so at 10 h.p.f., 24 h.p.f. and 1.5 d.p.f., P <0.005), but shisa2 contains only a single synonymous change between cave and surface fish. A duplicate copy of shisa2 is also under an eye QTL found on LG6 (refs 4 , 8 ), and this paralog exhibits no coding differences and elevated, but mostly non-significant, expression in cavefish (24 h.p.f., P <0.0003, not significant at 10 h.p.f. and 1.5 d.p.f.) and lower expression in cavefish at 3 d.p.f. ( P <0.0002). Because shisa2 interacts with major drivers of development, we further assessed quantitative and spatial differences of expression for the two shisa2 genes (LG2 and LG6) by quantitative PCR (qPCR) and in situ hybridization on Astyanax embryos. For both genes, qPCR experiments did not detect significant differences at 36 h.p.f. between the two morphs, suggesting an expression difference of less than twofold ( Fig. 3a ; Mann–Whitney U -test, P >0.05). At this stage, shisa2 -LG2 was expressed throughout the epidermis as well as in the olfactory epithelium and the lens in surface fish, but lens expression was notably missing in cavefish ( Fig. 3b ). Shisa2 -LG6 had a more complex expression pattern, reminiscent of what was described in Xenopus [37] and zebrafish [38] , and included expression in the branchial arches, cranial ganglia, epidermis, olfactory epithelium (like shisa2 -LG2), retina and lens ( Fig. 3c ). No obvious difference was observed between surface fish and cavefish embryos concerning shisa2 -LG6 expression pattern. In sum, anatomical analysis detected a lack of s hisa2 (LG2) expression in the cavefish lens, which suggests changes in the regulatory region of this gene may contribute to the loss of eyes in cavefish. 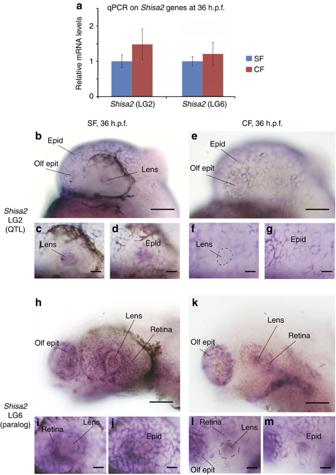Figure 3: Expression patterns ofshisa2. (a) Quantitative PCR forshisa2genes on 36 h.p.f. whole larvae of surface fish (blue) and cavefish (red). No significant difference was found between cavefish and surface fish expression (Mann–WhitneyU-test,P>0.05). The error bar is the s.e. of the mean, and the sample size is three in each case (each triplicate is a pool of 10–15 36 h.p.f. larvae). Photographs ofin situhybridization for the indicatedshisa2mRNA at 36 h.p.f. on surface fish (b–d,h–j) and cavefish (e–g,k–m) embryos, focusing on head and eye expression. The bottom pictures (c,d,f,g,i,j,l,m) are centered on the eye region, with focus either on the lens/retina or on the overlying skin. In all panels, anterior is left and dorsal is up. Inb,e,h,k, the photographs were taken from lightly labelled embryos (the epidermis is barely labelled) and inc,d,f,g,i,j,l,m, the photographs were taken from more strongly labelled embryos (epidermis expression is visible). Epid, epidermis; olf epit, olfactory epithelium (nose). The scale bars are 25 μm for panelsb,e,h,kand 10 μm for the other panels. Figure 3: Expression patterns of shisa2 . ( a ) Quantitative PCR for shisa2 genes on 36 h.p.f. whole larvae of surface fish (blue) and cavefish (red). No significant difference was found between cavefish and surface fish expression (Mann–Whitney U -test, P >0.05). The error bar is the s.e. of the mean, and the sample size is three in each case (each triplicate is a pool of 10–15 36 h.p.f. larvae). Photographs of in situ hybridization for the indicated shisa2 mRNA at 36 h.p.f. on surface fish ( b – d , h – j ) and cavefish ( e – g , k – m ) embryos, focusing on head and eye expression. The bottom pictures ( c , d , f , g , i , j , l , m ) are centered on the eye region, with focus either on the lens/retina or on the overlying skin. In all panels, anterior is left and dorsal is up. In b , e , h , k , the photographs were taken from lightly labelled embryos (the epidermis is barely labelled) and in c , d , f , g , i , j , l , m , the photographs were taken from more strongly labelled embryos (epidermis expression is visible). Epid, epidermis; olf epit, olfactory epithelium (nose). The scale bars are 25 μm for panels b , e , h , k and 10 μm for the other panels. Full size image In Xenopus embryos, s hisa2 morpholino knockdown or mRNA injection elicit the expression changes for otx2 , a key homeobox gene for head and eye development [36] . We, therefore, also compared otx2 expression patterns and levels in Astyanax cavefish and surface fish embryos, though we cannot localize this gene onto a specific LG. While otx2 pattern is similar in the two morphs during head and brain development ( Fig. 4b ), lens expression is much weaker in cavefish at 48 h.p.f. ( Fig. 4c ), as well as when assessed by whole-organism semi-quantitative reverse transcriptase-PCR ( Fig. 4a , Supplementary Fig. 2 ). We have, therefore, identified a potential developmental regulatory cascade that may lead to the cavefish eye loss and that would involve shisa2 and otx2 in the developing lens. 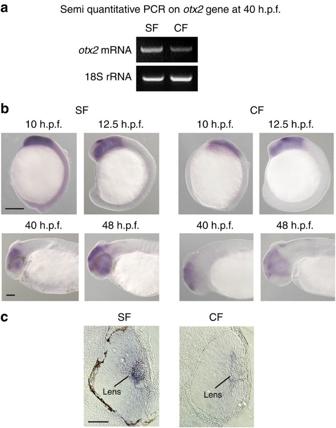Figure 4: Expression patterns ofotx2. (a) Semi-quantitative reverse transcriptase-PCR for theoxt2genes on 40 h.p.f. whole embryos. Cavefish (CF)otx2transcripts are slightly less abundant than those of surface fish (SF) compared with an 18S rRNA standard. (b) Photographs ofin situhybridizations forotx2mRNA at 10, 12.5, 40 and 48 h.p.f. on surface fish (SF) and CF embryos, focusing on head and eye expression. In all panels, anterior is on the left. In lower panels, dorsal is up. Scale bars are 100 μm for panels labelled 40 and 48 h.p.f. in (b). Scale bars are 250 μm for panels labelled 10 and 12.5 h.p.f. inb. (c) Sections ofin situ-hybridized SF and CF larvae at 48 h.p.f. show strongotx2downregulation in the cavefish lens. Scale bars are 100 μm for panels inc. Figure 4: Expression patterns of otx2 . ( a ) Semi-quantitative reverse transcriptase-PCR for the oxt2 genes on 40 h.p.f. whole embryos. Cavefish (CF) otx2 transcripts are slightly less abundant than those of surface fish (SF) compared with an 18S rRNA standard. ( b ) Photographs of in situ hybridizations for otx2 mRNA at 10, 12.5, 40 and 48 h.p.f. on surface fish (SF) and CF embryos, focusing on head and eye expression. In all panels, anterior is on the left. In lower panels, dorsal is up. Scale bars are 100 μm for panels labelled 40 and 48 h.p.f. in ( b ). Scale bars are 250 μm for panels labelled 10 and 12.5 h.p.f. in b . ( c ) Sections of in situ -hybridized SF and CF larvae at 48 h.p.f. show strong otx2 downregulation in the cavefish lens. Scale bars are 100 μm for panels in c . Full size image In addition to shisa2 , we identified candidate genes under this potentially pleiotropic QTL. Several genes meeting our criteria under this particular QTL include prox1 and AIFM1 . Two additional genes found in the QTL analysis of O’Quin et al . [15] , crxa and Tbx2a , are also present under this QTL in our analysis. Prox1 regulates many processes in development including lens fibre elongation and differentiation and the exit of retinal progenitor cells from the cell cycle reviewed in ref. 39 . The knockdown of prox1 results in the disruption of the lens-specific γ-crystallin expression and subsequent lens apoptosis [40] . Cavefish expression of prox1 exhibits a similar spatial pattern to surface fish in the developing lens, and for this reason prox1 was previously considered unlikely to play a role in the cave-specific eye degeneration [41] . Prox1 is expressed in sensory hair cells of the neuromast and taste receptor cells of taste buds, both of which are more numerous in cavefish relative to surface, but prox1 expression in these structures does not occur until 96 h.p.f. (ref. 41 ). We detected no sequence differences between cave and surface fish for prox1 . However, in our whole-organism RNAseq data, significantly lower expression in cavefish was observed at 24 h.p.f., 1.5 d.p.f. and 3 d.p.f. ( P <0.022 in all cases), while marginally non-significant higher expression in cavefish was observed at the earliest sampled time point (10 h.p.f., P =0.083). Significantly lower expression of prox1 during these developmental time points is consistent with increased lens apoptosis in cavefish. Therefore, a re-examination of the contribution of prox1 , in light of its location under this QTL for suborbital neuromast cell number, VAB and eye size [7] and its quantitative expression differences, may be warranted. AIFM1 is implicated in significant and progressive optic atrophy in mutant Harlequin mice, and this mutant phenotype can be rescued by injection of an expression vector containing AIFM1 (ref. 42 ). Cavefish exhibit significantly lower expression of AIFM1 at 24 h.p.f. ( P <0.003) than surface fish, and this gene exhibits an intronic splice region variant and five nonsynonymous variants, two of which appear derived in cavefish. These variants were all predicted to be tolerated by a computational method that attempts to determine if an amino acid substitution is detrimental to protein function (SIFT [43] ). Interestingly, the paralog of this gene, AIFM2 , is also located under the QTL for eye size found on LG14 (ref. 4 ) and LG4 (ref. 7 ). AIFM2 has significantly reduced expression in cavefish relative to surface fish at most time points (10 h.p.f., 24 h.p.f., 3 d.p.f. ; P <0.022 in all cases) with qualitatively lower expression at 1.5 d.p.f. ( P =0.095). Further, the two splice region variants are fixed between the surface and cavefish, one of which also results in a nonsynonymous change that is putatively derived in cavefish, though this change is predicted by SIFT to be tolerated. Crxa induces retinal stem cells to differentiate into functional photoreceptors [44] . When knocked down in zebrafish, crxa prompts the downregulation of genes in the phototransduction cascade [45] , and is implicated in eye reduction experienced by another troglomorphic fish, Sinocyclocheilus anophtalmus [46] . This gene exhibits significantly reduced expression in cavefish at 1.5 and 3 d.p.f. ( P <0.001; at the other time points, expression could not be tested). Crxa contained no sequence differences between cave and surface fish. Tbx2a exhibits localized expression in zebrafish mainly in the otic placode, optic vesicle, otic vesicle and retina (also in ventral mesoderm and pectoral fin bud) [38] . T bx2 results in smaller optic cups when mutated in mice [47] , and two copies exist in zebrafish. Tbx2a is involved in craniofacial and pharyngeal arch development [48] , and its paralog T bx2b is required for proper retinal neuronal formation in zebrafish [49] . Tbx2a exhibits lower expression in cavefish at all time points ( P <0.07 at 1.5 d.p.f., P <0.001 at all other time points) and three nonsynonymous differences between cave and surface. Only one nonsynonymous difference is putatively derived in cavefish (D401E), and such an amino acid replacement is predicted by SIFT to be tolerated. Under the second co-localizing QTL for the traits’ vibration attraction behaviour, superficial neuromast number at orbit and eye size located on LG17 in Yoshizawa et al . [7] , we lacked scaffold coverage for several markers in the center of the QTL (208e, 205d and 221a; Supplementary Data 17 ). There are several interesting genes in this region ( Supplementary Data 11 ), but few are as compelling as genes found on the co-localizing QTL on LG2 of Yoshizawa et al . [7] We expect future drafts of the genome to uncover additional candidate genes in this region. Candidate genes for additional cave phenotypes Lastly, we sought to briefly investigate other distinctive traits for cavefish, including reduced pigmentation [5] , [6] . First, we found that one of the most famous pigmentation genes, mc1r , known to be mutated in Pachón cavefish [5] (the population from which the QTL were mapped), is located under the critical region of the QTL for number of melanocytes in four regions of the body (LG9 (refs 4 , 8 )). Second, cavefish have an increased number of taste buds and increased number of maxillary teeth [4] , [8] . A QTL for number of taste buds contains the serotonin receptor htr2a (LG5 (refs 4 , 8 )), and taste cell development and signal transduction involves serotonin signalling [50] , [51] . Third, a QTL for the number of maxillary teeth in cavefish (LG13 (refs 4 , 8 )) contains dact2 , which significantly inhibits dlx2 during tooth formation in mouse [52] . When knocked out in mice, dlx2 produces a decrease in the number of molars [53] , supporting the notion that this gene may have a conserved role in the regulation of tooth formation. Analyses of putative gene losses We investigated genes that were putatively lost in the cavefish lineage since the divergence of cavefish and zebrafish, by examining genes that were present in zebrafish and eight additional actinopterygian teleosts available in Ensembl ( Supplementary Data 18 ). These genes were not enriched for 305 gene ontology accessions related to eye development or function, and similar results were obtained for ZFIN anatomical expression data and ZFIN-predicted phenotype. Transcriptome data from the eight tissues used for gene annotation and the developmental surface fish and cavefish time series were assembled using Trinity [54] for a total of 10 separate transcriptomes. Open reading frames were predicted from these assemblies using Transdecoder in the Trinity package. We constructed a BLAST database from the coding regions of zebrafish from Ensembl Genes 74 and queried this database using each of the transcripts in the longest_orfs.cds files with BLASTn. We used a strong e-value cutoff (cutoff<1E-100), and results were robust for all values we examined from 1E-20 to 1E-100. In this way, we identified whether the putatively missing gene in the cavefish genome (but present in the zebrafish genome) was potentially present in the surface or cave-derived RNAseq data. For several genes that were potential candidates for loss, we could not find a representative transcript for cavefish but could find a transcript copy among the surface fish transcriptome data ( Supplementary Data 19 ). We attempted to confirm the lack of a transcript in cavefish using reverse transcription. However, for all cases that we tried to confirm a putatively missing cavefish transcript, a cavefish transcript was detected. Although not adding evidence for cavefish-specific loss, for several large gene families, one or several members were not annotated in the genome sequence and were not detected in surface or cavefish transcriptome data. While these results are very preliminary, potential candidates for gene loss include members of gene families involved in vision such as retinol dehydrogenases, crystallins, sine oculis homeoboxes, opsins/rhodopsins (including melanopsin whose truncating mutation is implicated in the loss of a light-entrainable clock in Somalian cavefish [55] ), development, regulation of sleep and circadian clocks (including fibroblast growth factors, gamma-aminobutyric acid A receptors, and dopamine receptors). Likewise, cavefish exhibit excessive locomotor activity compared with surface fish [56] , and several genes that induce hyperlocomotion when knocked out or blocked in mice or zebrafish do not appear to be present in the current cavefish genome annotation or transcriptome data ( Supplementary Data 19 ). Interestingly, the naked mole rat, a species that also lives in darkness and has reduced eyes, has also experienced losses in similar gene families [57] . Assembly and annotation errors of large gene families are common in draft genomes; thus, a more extensive and definitive exploration of these complex gene families awaits future studies. We provide a list from the initial, preliminary analysis ( Supplementary Data 19 ) to facilitate future studies. In this work, we present a draft genome of the Mexican cavefish, Astyanax mexicanus and identify candidate genes for some of the species’ most iconic phenotypes. Past efforts have focused on mapping traits to genomic regions [4] , [7] , [8] , [9] , [10] , [15] . By leveraging these past studies, we demonstrate the utility of the genome for candidate gene discovery, and highlight several potential regulators of eye development that were previously not implicated in cavefish eye degeneration. We also analysed RNAseq data to identify coding variants between cavefish and surface fish and narrow the list of candidate genes that potentially impact degeneration of the eye. Identification of candidate genes from past QTL work is especially exciting in A. mexicanus because cavefish are amenable to a host of molecular genetic techniques that can be used to validate allelic effects (for example, injection of messenger RNA into developing embryo [13] , meganuclease- and transposase-based transgenesis [14] ) and additional experimental techniques can be accomplished using the close relative and laboratory model zebrafish [5] (for example, gene editing technologies such as TALENs). Thus, cavefish represent a powerful system for examining the genetic bases of evolutionary change, and we expect progress in candidate gene identification will be more efficient with the addition of the genome. While a candidate gene approach has strong potential in the cavefish system, our expression analyses highlight the discoveries enabled by a pathway approach. In one example, our analysis predicted the reduced-eye phenotype in cavefish relative to surface fish by utilizing the direction of expression within eye development pathways. Notably, this result was one of the most significant phenotypes predicted as a downstream phenotypic effect from our developmental gene expression time course of whole embryos ( Supplementary Data 13–16 ). Nonetheless, many databases, including the ones used in this study (Ingenuity Pathway Analysis (IPA)), contain only orthologues from human, mouse and rat, and approximately 89% of the genes (2013/2408) in our QTL data set contained matches in the IPA database. This underscores the need for future iterations of these databases to include nonmammalian model species (for example, zebrafish, Drosophila ) to increase homology matches and, therefore, enable pathway analysis for a large swath of organisms. We anticipate that this genomic resource will be coupled with one of the largest strengths of the system, the repeated evolution of similar cave-associated traits in independently derived cave populations [2] . Crosses between fish from different caves complement and restore certain cave-derived phenotypes (for example, rudimentary eyes) [23] ; thus, at least some of the genetic changes accounting for cave-associated traits are unique to each cave lineage [9] . In addition, surface populations provide a pool of standing genetic variation for the caves [58] , and the cavefish system offers an interesting system for studying adaptation in the face of gene flow [2] . To investigate these questions, ongoing work that is beyond the scope of this paper includes a population genomic effort from several cave and surface localities. To enhance these efforts, the cavefish genome will need to be anchored to a physical, chromosome-scale map. Work to produce a higher-quality draft using long-read technology and a genotyping-by-sequencing linkage map is currently underway. We expect that this upcoming, revised draft will further aid investigations of the impact of selection, drift, migration and genetic architecture in creating theses replicated phenotypes. In conclusion, the Astyanax genome presented here will allow for dissection of the genetic bases of constructive and degenerative traits that make the cavefish distinctive, will facilitate future studies investigating the paths of repeated evolution and may advance understanding of human maladies (for example, sleep disorders, congenital eye defects) for which the cavefish can serve as a powerful natural model system. Source material Source DNA was obtained from the Jeffery Lab. DNA was collected from heart, liver, spleen and gill of a single 7–year-old adult female cavefish (Pachón) using the Genomic-Tip Tissue Midi kits (Qiagen, Valencia, CA). RNA from eight tissues was extracted with RNA Lipid Midi kits and RNeasy kits (Qiagen). Animal use complied with ethical standards and was approved by The University of Maryland Institutional Animal Care and Use Committee protocol number R-12–53 to W.R. Jeffery. Genome sequencing and assembly Using a genome size estimate of 1.19 Gb, total raw sequence coverage of Illumina reads was ~95 × (short insert paired-end reads, 3, 8 and 40 kb mate-paired libraries, Supplementary Data 1 ). The combined sequence reads were assembled using ALLPATHS software [59] and the assembled coverage was 70 × . This draft assembly was referred to as Astyanax mexicanus 1.0.2. This assembly has been gap filled with a version of Image [60] , modified for large genomes and cleaned of contaminating contigs by performing a MegaBLAST [61] of the contigs against adapter, bacterial and vertebrate databases. Identifying locations of QTL in genome assembly Many markers overlapped between previously published QTL analyses, rendering it possible to compare coarse QTL locations across replicated maps [4] , [7] , [8] , [15] , [16] , even though LG names were not consistent between studies. Markers flanking the QTL were localized to scaffolds via best BLAST hit. Briefly, a combination of 689 RAD-tag sequences, microsatellite markers and cDNAs with linkage map positions [15] were aligned to the scaffolds using BLASTn. Astyanax mexicanus has a haploid chromosome number of 25 (ref. 62 ), and there were a total on 24 LGs represented by these markers ( Supplementary Fig. 1 ). All markers were required to have an e-value of 1E-20 except for a subset of microsatellite and cDNA markers where only the forward primer, reverse primer and sometimes the repeat motif sequence were available. For these microsatellites, word size was reduced to ‘7’, and hits were required to have an e-value of less than 1E-1 and identity of greater than 99%. Two cDNAs taken from Danio rerio were also allowed weaker identity (85% or greater) and an e-value cutoff of 1E-1. Only the top BLAST hit for each marker was recorded. Scaffolds that mapped to different LGs were excluded ( n =9). In the case where three or more markers mapped the scaffold to one LG and only a single marker mapped the scaffold to a different LG ( n =3), only the incongruent marker was excluded. In total, 340 scaffolds were localized to LGs representing 574 Mb of sequence ( Supplementary Data 17 ). Scaffolds with only a single marker (219 scaffolds) were ordered along the chromosome in line with the genetic map as described in ref. 15 and the orientation was assigned randomly. Orientation was assigned for scaffolds with two or more markers (121 scaffolds, ~339 Mb) physically and genetically mapped ( Supplementary Data 17 ; Supplementary Fig. 1 ). Such a map is very similar to what is given in the Supplementary Materials of ref. 9 . Repetitive landscape Repeats, including TEs, were identified and annotated using RepeatModeler software with default parameters. The annotation follows the universal classification [63] . The automatic library was screened to filter and discard sequences sharing high similarities with Uniprot protein. Parallel to the automatic annotation, potentially absent families that were not found using RepeatModeler were manually searched by BLAST using known TE proteins. The unplaced scaffolds were masked using RepeatMasker 3.3.0 ( http://www.repeatmasker.org/ ) with the cavefish-specific repeated library using ‘–lib’ and ‘–align’ functions. Results were parsed to determine copy number and coverage of TE superfamilies using the RepeatMasker outfiles. To investigate the level of TE transcription, we analysed three different assembled transcriptomes: muscle, brain and whole-eye surface fish. Transcriptomes were masked using RepeatMasker 3.3.0 using the specific cavefish repeat library, as was done for the genomic analyses. The proportion of the various classes (for example, DNA, LINE, SINE, LTR and unknown elements) were compared with their respective proportions in the genome (camembert graphs). We assayed for over- and under-representation of TE superfamilies by comparing the respective proportion of each family and superfamily in the genome and in the transcriptomes. The following equation was used: (percentage of the TE family in the genome [or transcriptome] * 100)/Total repeat content in the genome [or transcriptome]). Gene prediction and annotation Iterative steps that rely on similarity evidence from prior teleost gene models and ab initio gene prediction algorithms were followed to build gene models according to established methods at Ensembl [18] . Protein-coding models were extended into UTR regions and completed exon models were validated with RNAseq data (RNAseq analyses section below) from diverse tissue types. Additional methods followed here for generating gene builds by Ensembl are located at: http://useast.ensembl.org/info/genome/genebuild/2013_10_cavefish_genebuild.pdf . Although not used in these studies, a second gene set produced with the NCBI gene annotation pipeline is available at: ftp://ftp.ncbi.nlm.nih.gov/genomes/Astyanax_mexicanus/. RNAseq analyses RNAseq data was obtained from two different sequencing efforts. The first consisted of tissue-specific 100-bp paired-end Illumina reads which were used for genome annotation by Ensembl ( Supplementary Data 2 ). These included samples from brain, heart, kidney, liver, muscle, nasal cavity and skin from adult Pachón cavefish and eyes from adult surface fish from Texas. For all tissues, multiple (one to six) individuals were pooled, except for eyes where one surface individual was used. The second RNAseq sequencing effort consisted of a developmental time course of embryos taken from 10 h.p.f., 24 h.p.f., 1.5 d.p.f. and 3 d.p.f. Fifty individuals were pooled for each time point. Three separate TruSeq2 Illumina libraries were made for each time point from the same pool of RNA, providing technical replicates. Time-course RNAseq data were cleaned by trimming the first base with Fastx_trimmer ( http://hannonlab.cshl.edu/fastx_toolkit/ ), trimming with Trimmomatic v0.30 (ref. 64 ) using the adapter library for TruSeq2, allowing a quality score of 30 across a 4-bp sliding window and removing all reads <30 nucleotides in length after processing. Reads were aligned to the reference genome using TopHat2 (ref. 65 ) with default parameters except that the maximum intron length was set to 10,000. Cufflinks 2.1.0 (ref. 28 ) was used to calculate differences in expression between cave and surface RNAseq data. Cufflinks was used with the parameters: --frag-bias-correct --multi-read-correct --upper-quartile-norm --compatible-hits-norm (with the gtf file for the genome). Cuffdiff was used with the parameters: --frag-bias-correct --multi-read-correct --FDR 0.1 --dispersion-method per-condition. Time-course RNAseq work was performed under a protocol approved by the Institutional Animal Care and Use Committee (IACUC) of the University of Cincinnati; Protocol Number 10-01-21-01 to J.B.G. and complied with ethical regulation for treatment of animals. Samples for genome annotation were taken in the Jeffery lab under animal care protocols referenced above. Transcript variant analyses At most, 15 Pachón cavefish contributed to the offspring used in the RNAseq experiment (the same nine breeding individuals from Pachón Line 163 were used to generate embryos for 10 h.p.f., 24 h.p.f., 3 d.p.f. time points; six breeding individuals from Pachón Line 138 were used for 1.5 d.p.f.) and a total of three individuals contributed to the surface embryos from which RNAseq data were collected. These fish are laboratory stocks and likely somewhat inbred; thus, we had little power to assign allele frequencies between cave and surface pooled samples. For all analyses, we concentrate on differences that were completely fixed in our data set between the surface RNAseq genotypes and the cave reference genome+cave RNAseq genotypes. For variant calling, we concatenated all expression data for surface and separately concatenated all expression data for cave and mapped these ‘surface’ and ‘cave’ reads to the reference genome using TopHat2. These alignments were passed to Samtools v0.1.19 (ref. 66 ) to create mpileup files for cave and surface which were used by VarScan v2.3.6 (ref. 67 ) to call ‘somatic’ mutations with surface pileups designated as ‘normal’ and cave as ‘tumour.’ Variants were then used as input for Ensembl’s standalone Variant Effect Predictor v73 (ref. 68 ) to predict the class (for example, synonymous, nonsynonymous) of each variant. To determine if the substitutions identified by Variant Effect Predictor v73 were likely derived in cavefish, peptide sequence from orthologues of zebrafish, coelcanth, spotted gar, stickleback and platyfish were obtained from Biomart and aligned with ClustalW [69] . In most cases, it was straightforward to classify whether the surface or cave amino acid was likely derived, and in all other cases the site appeared evolutionarily labile. This analysis should be interpreted with the caveat that it does not account for the possibility that the variant classified as ‘derived’ in cavefish is actually present in the standing genetic variation of the surface fish which was not sampled in our data. SIFT Sequence was used to predict the functional impact of nonsynonymous substitutions [43] . Identification of candidate genes All pathway analyses were performed with the IPA suite of tools available at http://www.ingenuity.com/products/ipa . The entire ‘analysis-ready’ pool contained only 65% of genes in our QTL data set (1,560/2,408) ( Supplementary Data 12 ) as some of the genes under our QTL and in the IPA database did not have sufficient expression data for analysis. For all enrichment tests, we used only the analysis-ready gene set filtered by IPA, which does not include multiple genes with the same Entrez gene name or genes lacking expression data in our data set. In addition to the IPA analyses, which did not annotate all of the genes under the QTL, we conducted independent literature searches on genes and prioritized those that were (1) differentially expressed in at least one of the developmental time points; (2) contained at least one fixed nonsense or missense difference between cave and surface fish; or (3) exhibited expression in an eye-related structure during development of the zebrafish (ZFIN anatomical database) or had a gene ontology annotation or description related to eye, retina, lens or optic function. Quantitative PCR for shisa2 For the shisa2 in situ hybridization and qPCR experiments, laboratory stocks of A. mexicanus surface fish originated from San Solomon Spring, Balmorhea State Park, Texas. Cavefish from Pachón cave were obtained in 2004–2006 from the Jeffery laboratory at the University of Maryland, College Park, MD, and were since then bred in the GIF animal facility. Total RNA was extracted from 36 h.p.f. cavefish or surface fish embryos with TRIzol reagent (Invitrogen) followed by purification and DNase treatment with the Macherey Nagel NucleoSpin RNAII kit. RNA amounts were determined by the Nanodrop 2000c spectrophotometer (Thermo Scientific). Total RNA (1 μg) was reverse transcribed in a 20-μl final reaction volume using the High Capacity cDNA Reverse Transcription Kit (Life Technologies, Grand Island, NY, USA) with RNase inhibitor and random primers following the manufacturer’s instructions. Quantitative PCR was performed on a QuantStudio 12K Flex Real-Time PCR System with a SYBR green detection protocol. cDNA (3 ng) was mixed with Fast SYBR Green Master Mix and 500 nM of each primer in a final volume of 10 μl. The reaction mixture was submitted to 40 cycles of PCR (95 °C, 20 s; (95 °C, 1 s; 60 °C, 20 s) × 40) followed by a fusion cycle to analyze the melting curve of the PCR products. Negative controls without the reverse transcriptase were introduced to verify the absence of genomic DNA contaminants. Primers were designed by using the Primer-BLAST tool from NCBI and the Primer Express 3.0 software (Life Technologies). Primers were defined either in one exon and one exon–exon junction or in two exons spanned by a large intron. Specificity and the absence of multi-locus matching at the primer site were verified by BLAST analysis. The amplification efficiencies of primers were generated using the slopes of standard curves obtained by a four-fold dilution series. Amplification specificity for each real-time PCR reaction was confirmed by analysis of the dissociation curves. Determined C t values were then exploited for further analysis, with the Gapdh and Actb1 genes as references. Each sample measurement was made at least in duplicate. Primer sequences for LG6- shisa2 were 0974-AM-LG6-F1 5′- CGCAGTGCCCATCTACGTG -3′ and 0975-AM-LG6-R1 5′- TGTTTGGGTCGCAGACAGC -3′. For LG2- shisa2 , the primer sequences were 0982-AM-LG2-F3 5′- GGGCACCACAGTTTTTCCAA -3′ and 0983-AM-LG2-R3 5′- CTGTCCGTGTGCCTGACTGA -3′. For Gapdh and Actb1 , primers were 0970-AMgapdh-F1 5′- GTTGGCATCAACGGATTTGG -3′ and 0971-AMgapdh-R1 5′- CCAGGTCAATGAAGGGGTCA -3′ and 0972-AMactb1-F2 5′- GCCATCATGCGTCTTGACCT -3′ and 0973-AMactb1-R2 5′- ATCTCACGCTCAGCGGTTGT -3′, respectively. For shisa2 work, animals were treated according to the French and European regulations for handling of animals in research. Authorization for use of animals for this work was provided by Paris Centre-Sud Ethic Committee (authorization number 2012-0052) to S.R. (number 91–116). Quantitative PCR for otx2 Total RNA was isolated from 40 h.p.f. surface fish and Pachón cavefish larvae using TRIzol (Life Technologies). cDNA was synthesized using the SuperScriptTM III First-Strand Synthesis Super Mix Kit and oligo (dT) 20 primers (Life Technologies). For semi-quantitative reverse transcriptase-PCR, part of the otx2 coding region was amplified from cDNA with primers 5′- ATGATGTCGTATCTCAAGCAACC -3′ (forward) and 5′- TAATCCAAGCAGTCGGCGTTGAAG -3′ (reverse) using PCR Master (Roche Applied Science, Indianapolis, IN, USA), which yielded an otx2 PCR product of 857 bp. The PCR cycling conditions were: one cycle of initial denaturation at 94 °C for 5 min, followed by 35 cycles of denaturation (94 °C for 30 s), annealing (58 °C for 30 s) and elongation (72 °C for 45 s) and a final elongation step at 72 °C for 7 min. Amplification of the control 18S rRNA was carried out using 1 μl of the synthesized cDNA with primers in a 50-μl reaction volume using PCR Master (Roche). The 18S rRNA primers were 5′- GAGTATGGTTGCAAAGCTGAAA -3′ (forward) and 5′- CCGGACATCTAAGGGCATCA -3′ (reverse), which yielded a PCR product of 343 bp. The PCR cycling conditions were: one cycle of initial denaturation at 94 °C for 5 min, followed with 25 cycles of denaturation (94 °C for 30 s), annealing (at 62 °C for 30 s) and elongation (at 72 °C for 30 s), followed by a final elongation step at 72 °C for 7 min. Whole-mount in situ hybridization for shisa2 cDNAs were amplified by PCR from pCMV-Sport6 plasmids picked from our cDNA library using SP6 and T7 primers and digoxygenin-riboprobes were synthesized from PCR templates. A protocol for automated whole-mount in situ hybridization (Intavis) was performed. Briefly, embryos were progressively rehydrated, permeabilized by proteinase K (Sigma) treatment before being incubated overnight at 68 °C in hybridization buffer containing the appropriate shisa2 probe. After stringent washes, the hybridized probes were detected by immunohistochemistry using an alkaline phosphatase-conjugated antibody against digoxygenin (Roche) and a NBT/BCIP chromogenic substrate (Roche). Whole-mount in situ hybridization for otx2 For probe preparation, the otx2 coding region fragment was amplified from surface fish cDNA with PCR Master (Roche) according to the ‘Hot start’ PCR protocol using the otx2 primers described above. The PCR cycling conditions were: one cycle of initial denaturation (94 °C) for 2 min, followed by 32 cycles of denaturation (94 °C for 30 s), annealing (58 °C for 30 s) and elongation (72 °C for 45 s) and a final elongation step (72 °C for 7 min). The first PCR product was used as the template for a second cycle of PCR amplification using same conditions. The resulting 857 bp PCR product was cloned into the TOPO vector in the TPO TA Cloning Kit Dual Promotor (Life Technologies) and confirmed by sequencing. In situ hybridization was performed according to ref. 70 with some modifications. The plasmid DNA was linearized with restriction enzymes Bam H 1 and Xho I (Life Technologies) at 37 °C for 1 h and purified with the QIAquick PCR Purification Kit (Qiagen). Sense and antisense digoxigenin (DIG)-labelled RNAs were transcribed with SP6 RNA and T7 RNA Polymerases (Roche). The in vitro transcription reactions were conducted according to the DIG RNA Labeling Mix (Roche) protocol. The reactions were terminated with 0.2 M EDTA (pH 8.0), and RNA was precipitated with 4 M LiCl and washed in prechilled 70% ethanol. The RNA probe was denatured for 3 min at 95 °C, quickly cooled on ice for 5 min and then added to the HYB+ (see below) to obtain a concentrated stock (10 μg ml −1 ). The embryos were fixed with 4% paraformaldehyde in PBS overnight at 4 °C, dehydrated in an increasing methanol series and stored at −20 °C. Rehydrated embryos were treated with proteinase K (10 μg ml −1 in PBST (PBS plus 0.1% Tween 20)) for 5–10 min at room temperature, washed twice with PBST, post fixed for 20 min with 4% paraformaldehyde in PBST and washed 5 times with PBST (5 min each). The embryos were pretreated with HYB− (50% formamide, 5 × SSC, 0.1% Tween 20) for 5 min at 60 °C without shaking. The HYB− was replaced with HYB+ (HYB−, 1 mg ml −1 yeast RNA, 50 μg ml −1 heparin) and the embryos were prehybridized at 60 °C for 4 h with gentle shaking. The prehybridization mix was removed and replaced with 1 ng μl −1 of otx2 sense or antisense probe in HYB+. Hybridization was carried out at 60 °C overnight with gentle shaking. The embryos were then washed twice at 60 °C with 50% formamide/2 × SSCT (saline sodium citrate plus 0.1% Tween 20) for 30 min each, once with 2 × SSCT for 15 min at 60 °C, twice with 0.2 × SSCT (20 min each) at 60 °C and twice with MABT (150 mM maleic acid, 100 mM NaCl, pH7.5, 0.1% Tween 20) for 5 min each at room temperature. The embryos were incubated with blocking solution (MABT, 2% blocking reagent) overnight at 4 °C with rocking and then with Anti-DIG-AP Fab fragments (1:5,000; Roche) in blocking solution overnight at 4 °C with gentle rocking. The embryos were washed once with MABT containing 10% sheep serum at room temperature for 25 min and eight more times (45–60 min each) with MABT at room temperature with gently shaking. Then, the embryos were washed with PBST and incubated in BM Purple AP Substrate (Roche) at room temperature in the dark. After the signal developed, the reaction was terminated by rinsing the embryos several times in PBST. Embryos were processed through an increasing glycerol series in PBS (30–50–80%) and imaged by microscopy. In situ -hybridized embryos were dehydrated through an ethanol series (from 30, 50, 70, 85, 95%, and three 100% steps) for 20 min each at room temperature. The dehydrated embryos were incubated in ethanol:Histo-Clear (1:1) with rotation for 20 min, in two changes of Histo-Clear for 30 min each), in paraffin:Histo-Clear (1:1) at 62 °C for 1 h and finally 100% paraffin at 62 °C for 2 h. The blocks containing embedded embryos were cut into 15-μm sections, and the sections were dewaxed and viewed by microscopy. How to cite this article : McGaugh S. E., et al . The cavefish genome reveals candidate genes for eye loss. Nat. Commun. 5:5307 doi: 10.1038/ncomms6307 (2014). Accession codes: All genomic data are associated with bioproject PRJNA89115 and have been deposited in GenBank/EMBL/DDBJ Nucleotide database under the accession code APWO00000000. RNAseq data have been deposited in the GenBank/EMBL/DDBJ sequence read archive under the accession codes PRJNA177689 (tissue-specific transcriptomes) and PRJNA258661 (developmental time course). Gene annotations can be found at http://www.ensembl.org/Astyanax_mexicanus/Info/Index and have been deposited in the GenBank/EMBL/DDBJ Assembly database under the accession code PRJNA237016 .